A low-nuclear Ag4nanocluster as a customized catalyst for the cyclization of propargylamine with CO2 The preparation of 2-Oxazolidinones using CO 2 offers opportunities for green chemistry, but multi-site activation is difficult for most catalysts. Here, A low-nuclear Ag 4 catalytic system is successfully customized, which solves the simultaneous activation of acetylene (-C≡C) and amino (-NH-) and realizes the cyclization of propargylamine with CO 2 under mild conditions. As expected, the Turnover Number (TON) and Turnover Frequency (TOF) values of the Ag 4 nanocluster (NC) are higher than most of reported catalysts. The Ag 4 * NC intermediates are isolated and confirmed their structures by Electrospray ionization (ESI) and 1 H Nuclear Magnetic Resonance ( 1 H NMR). Additionally, the key role of multiple Ag atoms revealed the feasibility and importance of low-nuclear catalysts at the atomic level, confirming the reaction pathways that are inaccessible to the Ag single-atom catalyst and Ag 2 NC. Importantly, the nanocomposite achieves multiple recoveries and gram scale product acquisition. These results provide guidance for the design of more efficient and targeted catalytic materials. The conversion of CO 2 into high-value-added chemicals [1] , [2] , [3] , [4] , [5] , [6] , [7] , such as starch [8] , carboxylic acid [9] , [10] , propylene carbonate [11] , [12] , and 2-oxazolidinone [13] , is considered a promising approach to achieve carbon neutrality and has become a hot topic in the field of catalysis. In particular, 2-oxazolidone compounds have important application potential in organic intermediates, antibacterial drugs and chiral auxiliaries [14] , [15] . Ideally, the greenest preparation of 2-oxazolone compounds is the cyclization of propargylamine with CO 2 . However, due to the unique structure of propargylamine, which contains both acetylene (-C≡C) and amino (-NH-) functional groups, it is difficult for most current catalysts to achieve this transformation [16] , [17] , [18] , [19] . Therefore, there is an urgent need to customize a catalyst with multiple active sites for the cyclization of propargylamine with CO 2 . Single-atom catalysts (SACs) have been widely used for CO 2 conversion due to their high molar utilization, clear active site, and unique electronic structure [20] , [21] , [22] , [23] . However, the presence of only a single metal site inherently limits SACs performance [24] , [25] , [26] , [27] , [28] . In contrast, low-nuclear nanoclusters (NCs) not only show the same characteristics as SACs but also benefit from synergistic effects between adjacent metals [29] , [30] , [31] , [32] , [33] , [34] , [35] , [36] . However, low-nuclear-weight NCs are more prone to unpredictable structural transformations under harsh environments [37] , [38] , making it difficult to identify the true active component. Scott et al. reported that alkyne-protected Cu 20 NC do not require harsh pretreatment during catalysis [39] , Wang et al. reported that an alkyne-protected Au 38 NC exhibited superior performance compared to that of a sulfate-protected Au 38 NC [40] . Zheng et al. found that the activity of intact Au 34 Ag 28 (PhC≡C) 3 is significantly better than that of partially or completely removed ligands [41] . Alkyne ligands, as metal-organic ligands, are considered to play an important role in improving the catalytic performance [42] , [43] , [44] . Therefore, we designed a low-nuclear Ag 4 NC protected by alkynes for the cyclization of propargylamine with CO 2 . As expected, the customized Ag 4 NC achieved the highest TON value of 5746.2, significantly higher than that of reported catalysts and the corresponding Ag 2 NC, Ag 6 NC and Ag 9 NC. Moreover, three Ag 4 *NC intermediates were captured and confirmed their structures by ESI and 1 H NMR. The key role of four Ag atoms revealed the feasibility and importance of low-nuclear catalysts at the atomic level. More importantly, the obtained Ag 4 /TNT nanocomposite afforded the product at the gram scale. A low-nuclear alkyne-protected Ag 4 NC and the corresponding Ag 6 NC and Ag 9 NC were synthesized according to the literatures [45] , [46] , [47] . All these Ag NCs were characterized by mass spectrometry, UV‒vis absorption spectroscopy, and single-crystal diffraction analysis (Fig. 1a and Supplementary Figs. S1 – S3 ), confirming the atomic monodispersity and the exact formula assigned to Ag 4 NC, Ag 6 NCand Ag 9 NC, respectively. N-Benzylprop-2-yn-1-amine ( 1a , HC≡CCH 2 NHBn) was selected as the preferred substrate for the cyclization of propargylamine to explore the catalytic performance of the customized Ag 4 NC. As expected, the Ag 4 NC protected by the acetylene ligand showed the best performance. To exclude the influence of the number of metal atoms, we designed and synthesized Ag 2 NC through a controlled experiment and compared their activity (Fig. 1a and Supplementary Fig. 4 ). Interestingly, among the Ag n ( n = 2,4,6,9) NC series, Ag 4 NC had the highest catalytic activity with TON and TOF values up to 5746.2 and 2873.1 h −1 , respectively, which were higher than those of reported catalysts (Fig. 1b and Supplementary Table 3 ). Then, we investigated the catalytic activity of AgNO 3 , AgBF 4 and [Ag(C≡C t Bu)] n , and the results show that the activity of these catalysts is low. 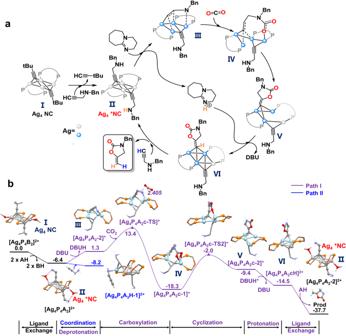Fig. 3: Proposed mechanism and calculation of the relative Gibbs free energies for Ag4NC. aProposed mechanism by Ag4NC.bThe relative Gibbs free energies, in bold. Gibbs free energy profiles of the Ag4NC on carboxylation of N-benzylprop-2-yn-1-amine. Abbreviated labels: AH (N-benzylprop-2-yn-1-amine,1a); BH (3,3-Dimethyl-1-butyne); c(CO2); P2(dppf). For clarity, the two MeOH molecules, all H atoms (unless the reaction site), and the benzyl group on N-benzylprop-2-yn-1-amine were omitted in all structures except for Ag4P4B2and Ag4P4A2. Silver: silver and light blue. 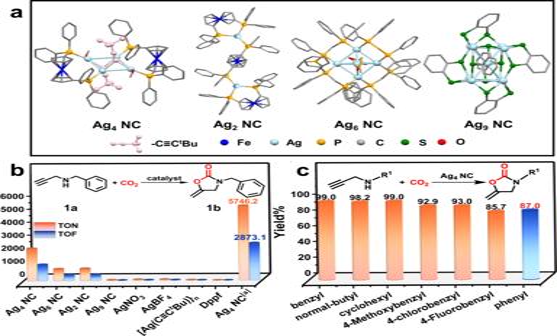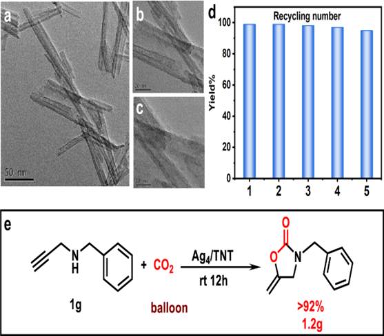Fig. 4: Characterization and applications of Ag4/TNT. a–cTEM images of Ag4/TNT.dRecoverability of Ag4/TNT catalysts in the cyclization of propargylamine with CO2. reaction conditions: Ag4/TNT (50 mg, 1.6 wt% loading of NCs), N-benzylprop-2-yn-1-amine (0.5 mmol), DBU (0.05 mmol), acetonitrile (1.0 mL), 25 °C, 12 h, CO2balloon.eGram scale experiment. Furthermore, the Ag 4 NC with a Dppf (1,1’-Bis(diphenylphosphino)ferrocene) ligand was inactive for this reaction (Fig. Fig. 1: Activity comparison and substrate expansion. aTotal structure of the Agn(n= 2,4,6,9) NCs.bTON and TOF value of different catalysts for CO2cycloaddition of N-benzylprop-2-yn-1-amine. Reaction conditions: Ag4NC (0.04 mol%), propargylamine (0.5 mmol), DBU (0.05 mmol), solvent (1 mL), 25 °C and CO2balloon. Yields and selectivity were determined by gas chromatography. [a] propargylamine (1.5 mmol), DBU (0.15 mmol), solvent (1 mL), 25 °C and CO2balloon.cThe cyclization of various propargylamine with CO2. 1b and Supplementary Table 1 ). The changes in the kinetics of the cyclization of N-benzylprop-2-yn-1-amine with CO 2 catalyzed by low-nuclear Ag 4 NC were monitored by in situ 1 H NMR (Supplementary Fig. 5a ). 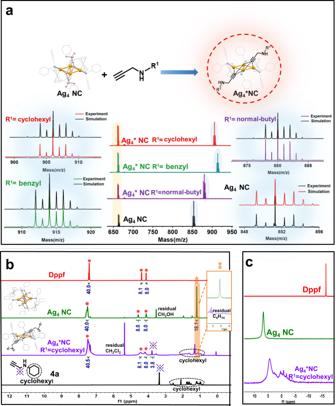Under the ideal conditions, we further explored the generality of the reaction for various propargylamine substrates. As shown in Fig. Fig. 2: Characterization of Ag4NC and Ag4* NC. aESI-MS spectra of the intermediate Ag4* NC and simulation of the corresponding mass spectrum.b1H NMR spectra of4a, Ag4* NC R1= cyclohexyl, Ag4NC, and Dppf.∗in red (Characteristic hydrogen of Dppf) ※ in purple (Characteristic hydrogen of the methylene group of N-2-Propyn-1-ylcyclohexanamine) ⁑ in orange (The methyl hydrogen peak (1.11 ppm) of the C≡CtBu ligand disappears.)c31P NMR spectra of Ag4* NC R1= cyclohexyl, Ag4NC, and Dppf. 1c and Supplementary Table 2 , Ag 4 NC afforded the target products in high yields within 2 h for all propargylamine substrates ( 3a-4a ) with alkyl terminations. Moreover, Ag 4 NC also reacted satisfactorily and afforded the corresponding products for substrates ( 5a-7a ) with either electron-withdrawing or electron-donating groups. Most studies have reported that the low nucleophilicity of substrates such as N-phenylpropyl-2-yn-1-amine ( 2a ) prevents the nucleophilic attack of carbon dioxide due to the benzene ring, resulting in a carbamate intermediate that is difficult to convert smoothly or requires high temperature conditions [16] , [48] . Much to our surprise and delight, the customized Ag 4 NC achieved highly active conversion of the N-phenylpropyl-2-yn-1-amine substrate at room temperature with yields up to 87%. Fig. 1: Activity comparison and substrate expansion. a Total structure of the Ag n ( n = 2,4,6,9) NCs. b TON and TOF value of different catalysts for CO 2 cycloaddition of N-benzylprop-2-yn-1-amine. Reaction conditions: Ag 4 NC (0.04 mol%), propargylamine (0.5 mmol), DBU (0.05 mmol), solvent (1 mL), 25 °C and CO 2 balloon. Yields and selectivity were determined by gas chromatography. [a] propargylamine (1.5 mmol), DBU (0.15 mmol), solvent (1 mL), 25 °C and CO 2 balloon. c The cyclization of various propargylamine with CO 2 . Full size image On this basis, we conducted relevant control experiments to gain more insight into the fundamental source of the catalytic activity of Ag 4 NC. The characteristic UV peak of Ag 4 NC showed a slight blueshift (8 nm) after Ag 4 NC was mixed with substrate 1a (1:2) for 1 h. In contrast, the characteristic peak of Ag 4 NC did not change at all within 2 h (Supplementary Fig. 5a ). The adsorption of 1a on the Ag 4 NC was detected by Fourier Transform Infrared (FT-IR) Spectroscopy. As shown in Supplementary Fig. 5c , the dominant stretching peak of C≡C-H at 3290 cm −1 disappeared, and the peak of C≡C at 2106 cm −1 shifted to 2120 cm −1 . This reveals that the H atom of C≡C-H was removed from 1a and that the C≡C bond of 1a was activated by Ag 4 NC, which was related to the dehydrogenation activation of 1a [49] . To obtain direct evidence of the interaction between Ag 4 NC and 1a , we captured the Ag 4 * NC intermediate by ESI-MS. As shown in Fig. 2a , the mass spectrum peaks of Ag 4 * NC (R 1 = benzyl) were detected and calculated to be 661.0 m/z and 914.0 m/z (Simulation: 661.3 m/z = [Ag+Dppf] + , 914.3 m/z = [1/2Ag 4 -C≡C t Bu + C≡CCH 2 NHBn-CH 3 OH] + respectively). The ESI-MS peaks of Ag 4 * NC (R 1 = benzyl) corresponded exactly to those of Ag 4 NC (661.3 m/z and 851.3 m/z, Simulation: 661.3 m/z = [Ag+Dppf] + , 851.3 m/z = [1/2Ag 4 -CH 3 OH] + , respectively). Notably, Ag 4 * (R 1 = benzyl) species were also successfully detected by ESI-MS in the reaction solution (Ag 4 + 1a + CO 2 ), suggesting that Ag 4 * NC is a key intermediate in the catalytic cycle (Supplementary Fig. 6a ). To confirm this hypothesis, we isolated and verified the activity of Ag 4 * NC (R 1 = benzyl). The experimental results showed that the activity of Ag 4 * NC and Ag 4 NC was similar, confirming that Ag 4 * NC was the key intermediate. The isolated Ag 4 * NC (R 1 =cyclohexyl), Ag 4 NC, dppf ligand and substrate 4a were characterized by 1 H NMR (Fig. 2b ). The 1 H NMR spectrum of Ag 4 NC contains the characteristic peak attributed to the hydrogen of the dppf and tert-butylvinyl ligands, and the ratio of the intensities of the peaks attributed to the benzene ring hydrogen (7.49 ppm) on the dppf ligand to the metal ring hydrogen (4.49 ppm, 4.03 ppm) and the C≡C t Bu ligand methyl hydrogen (1.11 ppm) was 40:8:8:18, and some peak shifts were observed. This was consistent with the molecular formula of Ag 4 NC, which reflects the structural integrity and high matching of the Ag 4 NC. Compared with the 1 H NMR spectrum of 4a , the 1 H NMR spectrum of Ag 4 * NC showed shifts in the characteristic peak of the hydrogen of the cyclohexyl group (marked by the black dashed circle) and the methylene hydrogen peak (purple symbol) in the substrate HC≡CCH 2 NHCy ( 4a ), while the methyl hydrogen peak of the C≡C t Bu ligand (1.11 ppm) disappeared. Additionally, the ratio of the intensities of the peaks attributed to the methylene hydrogen of C≡CCH 2 NHCy (3.69 ppm), the monocyclic hydrogen of the dppf ligand (4.10 ppm, 4.34 ppm) and the benzene ring hydrogen (7.40 ppm) was 3.8:8:8:40.5, indicating that the structure of the Ag 4 * NC molecule was similar to that of the Ag 4 NC molecule, including two dppf ligands and two C≡CCH 2 NHCy ligands. At the same time, it can be seen from the 31 P spectrum (Fig. 2c ) that the structure of Ag 4 * NC is similar to that of Ag 4 NC, and there is no free P ligand in the system. Moreover, the other substrates [HC≡CCH 2 NHCy ( 4a , R 1 = cyclohexyl) and HC≡CCH 2 NH n Bu ( 3a , R 1 = normal-buty)] were selected for the primitive reaction with Ag 4 NC. The ESI-MS results showed two ionic peaks located at 661.0 m/z and 906.0 m/z (Simulation: 661.3 m/z = [Ag+Dppf] + , 906.3 m/z = [1/2Ag 4 -C≡C t Bu+C ≡ CCH 2 NHCy-CH 3 OH] + , respectively), along with peaks at 661.0 m/z and 880.0 m/z (Simulation: 661.3 m/z = [Ag+Dppf] + , 880.3 m/z = [1/2Ag 4 -C≡C t Bu + C≡CCH 2 NH n Bu-CH 3 OH] + , respectively). Meanwhile, the Ag 4 * (R 1 = cyclohexyl) species was also successfully identified in the reaction solution (Ag 4 + 4a + CO 2 ) (Fig. 2a and Supplementary Fig. 6b ). Fig. 2: Characterization of Ag 4 NC and Ag 4 * NC. a ESI-MS spectra of the intermediate Ag 4 * NC and simulation of the corresponding mass spectrum. b 1 H NMR spectra of 4a , Ag 4 * NC R 1 = cyclohexyl, Ag 4 NC, and Dppf. ∗ in red (Characteristic hydrogen of Dppf) ※ in purple (Characteristic hydrogen of the methylene group of N-2-Propyn-1-ylcyclohexanamine) ⁑ in orange (The methyl hydrogen peak (1.11 ppm) of the C≡C t Bu ligand disappears.) c 31 P NMR spectra of Ag 4 * NC R 1 = cyclohexyl, Ag 4 NC, and Dppf. Full size image Consistent with the experimental observations, the ligand exchange of 3,3-dimethyl-1-butyne (BH) with N-benzylprop-2-yn-1-amine (AH) was found to be thermodynamically feasible (exergonic by 6.4 kcal/mol, Fig. 3b ). After that, two main types of mechanisms, depending on whether carboxylation occurs on the incoming A substrate (via ligand exchange, Path I) or an extra AH substrate (Path II, Supplementary Fig. 15 and Fig. 3b ), were investigated. In path I, the coordinated A group on Ag 4 P 4 A 2 first reacted with DBU, and this step was slightly endergonic by 7.7 kcal/mol (Fig. 3b ). Thereafter, carboxylation with CO 2 occurred on Ag 4 P 4 A 2 -2 to generate the intermediate Ag 4 P 4 A 2 c-1 (c represents CO 2 ), with a low activation barrier of 12.1 kcal/mol owing to the high nucleophilicity of the deprotonated amino group. Subsequent cyclization then occurred with a barrier of 16.3 kcal/mol. The resulting intermediate Ag 4 P 4 A 2 c-2 then underwent protonation and ligand exchange to complete the catalytic cycle. Overall, the Ag 4 -catalyzed cycloaddition of N-benzylprop-2-yn-1-amine was highly exergonic by -37.7 kcal/mol, and the carboxylation step was the rate-determining step (Ag 4 P 4 A 2 -2 → Ag 4 P 4 A 2 c-1). Path II started with the coordination of an extra AH substrate, preferentially via an amino group, to form Ag 4 P 4 A 3 H-1 (Supplementary Figs. 15 , 16 and Fig. 3b ). Similar to the overall transformation in Path I, deprotonation, carboxylation, cyclization, and protonation then occurred to generate the final product. However, the overall energy demands for Path II were 4.4 kcal/mol higher than those for Path I (26.0 vs. 21.6 kcal/mol in Fig. 3b and Supplementary Fig. 15 ). Of note, in this study, some other pathways, including deprotonation and carboxylation on Ag 4 P 4 A 3 H-1, were also examined but were excluded because of their relatively high energy demands (Supplementary Fig. 17 ). In this context, Path I was the most feasible pathway. Moreover, the carboxylation process of path I was experimentally investigated by 13 C NMR and ESI-MS. As shown in Supplementary Fig. 19 , the 13 C NMR carbon spectrum shows that the characteristic peaks of raw material 1a gradually weakened with the insertion of carbon dioxide. Meanwhile, new peaks assigned to the products gradually emerge and enhance. The characteristic peak signal changed significantly within 0.5 h, so we monitor the ESI-MS spectrum of the reaction solution during this period. To be noted, intermediate species IV (Fig. 3 ) was successfully detected by ESI-MS when Ag 4 NC, 1a and CO 2 were mixed for 15 min. The mass peak of [Ag 4 C≡CCH 2 NHBnC=CCH 2 CH 2 O 2 NBn (Dppf) 2 ] + was detected at 1871.6 m/z (simulation: 1871.6 m/z) (Supplementary Fig. 20 ), coincident with the species IV on path I of DFT calculations (Fig. 3b , via ligand exchange). The tetranuclear Ag 4 core was pivotal in stabilizing the deprotonated amino group in Ag 4 P 4 A 2 -2 and the anionic carboxylic group in Ag 4 P 4 A 2 c-1. Such an interaction was unlikely in the Ag 2 system, as Ag-N coordination resulted in remarkable structural distortion in the diphosphine ligand. This was also the reason the yield of the Ag 2 system was significantly lower than that of the Ag 4 system (Supplementary Fig. 18 ). Based on the above, we proposed a mechanism for the cyclization of propargylamine with CO 2 catalyzed by Ag 4 NC (Fig. 3a ). Obviously, Ag 4 NC first interacted with the propylamine substrate to produce the dehydrogenation activation product Ag 4 * NC, which remained in the form of Ag 4 * NC after cyclization. Throughout the catalytic process, activation of the substrate required coordination between multiple Ag atoms (the blue atoms represent the active Ag atoms), confirming the reaction pathways that are inaccessible to the Ag single-atom catalyst and Ag 2 NC. Fig. 3: Proposed mechanism and calculation of the relative Gibbs free energies for Ag 4 NC. a Proposed mechanism by Ag 4 NC. b The relative Gibbs free energies, in bold. Gibbs free energy profiles of the Ag 4 NC on carboxylation of N-benzylprop-2-yn-1-amine. Abbreviated labels: AH (N-benzylprop-2-yn-1-amine, 1a ); BH (3,3-Dimethyl-1-butyne); c(CO 2 ); P 2 (dppf). For clarity, the two MeOH molecules, all H atoms (unless the reaction site), and the benzyl group on N-benzylprop-2-yn-1-amine were omitted in all structures except for Ag 4 P 4 B 2 and Ag 4 P 4 A 2 . Silver: silver and light blue. Full size image To understand its applicability, the Ag 4 /TNT nanocomposite was successfully synthesized, which characterized by solid-state UV, XRD, TEM, XPS and element mapping (see Fig. 4 and Supplementary Figs. 7 – 11 for details). The Ag 4 /TNT nanocomposites demonstrated the same activity as Ag 4 NC, while TNT carrier was inactive (Supplementary Fig. 12 ). In this scenario, a recycling experiment was performed with 1a as the substrate, and the reaction efficiency did not show significant changes even after five runs (Fig. 4d and Supplementary Fig. 13 ). To determine the practicability of this transformation, a scale-up experiment afforded 3-benzyl-5-methylene-2-oxazolone in 1.2 g and >92% yield, which is comparable to previous results (Fig. 4e ). Fig. 4: Characterization and applications of Ag 4 /TNT. a – c TEM images of Ag 4 /TNT. d Recoverability of Ag 4 /TNT catalysts in the cyclization of propargylamine with CO 2 . reaction conditions: Ag 4 /TNT (50 mg, 1.6 wt% loading of NCs), N-benzylprop-2-yn-1-amine (0.5 mmol), DBU (0.05 mmol), acetonitrile (1.0 mL), 25 °C, 12 h, CO 2 balloon. e Gram scale experiment. Full size image In summary, alkyne-protected low-nuclear Ag 4 nanocluster (NC) is designed to catalyze the cyclization of propargylamine with CO 2 . As expected, the low-nuclear Ag 4 NC achieves the highest TON value of 5746.2, significantly higher than that of reported catalysts and the corresponding Ag 2 NC, Ag 6 NC and Ag 9 NC. In addition, the Ag 4 NC successfully achieves the cyclization of propargylamine with CO 2 under mild conditions. In the elementary reaction of Ag 4 NC with substrates, including HC≡CCH 2 NHBn, HC≡CCH 2 NHCy and HC≡CCH 2 NH n Bu, we capture three Ag 4 * NC intermediates and confirm their structures by Electrospray ionization (ESI). Density functional theory (DFT) calculations further confirm the key role of four Ag atoms, revealing the feasibility and importance of low-nuclear catalysts at the atomic level. Importantly, the Ag 4 /TNT (functional titanate nanotubes) nanocomposite afford the product at the gram scale. Therefore, the customized Ag 4 catalyst improves the reaction activity while exerting the atomic economy similar to that of single atom catalyst, which has advantages in reducing cost. The present work provides a new perspective on the mechanism of the cyclization of propargylamine with CO 2 , which provides further support for the design of further atomic level catalysts and their efficient utilization. Characterizations The UV−vis. spectra were recorded on a Techcomp UV 1000 spectrophotometer. Transmission electron microscopy (TEM) was conducted on a JEM-2100 microscope with an accelerating voltage of 200 kV. The FT-IR spectra were recorded with a Bruker Tensor 27 instrument. The X-ray diffraction (XRD) patterns were obtained on Smart Lab 9 KW with Cu Kα radiation. The NCs loaded on the TNT catalyst support were determined by Inductively Coupled Plasma Mass Spectrometry (ICP-MS). The X-ray photoelectron spectroscopy (XPS) measurements were conducted on ESCALAB 250Xi. Electrospray ionization mass spectra (ESI-MS) were recorded using a Waters UPLC H-class/Xevo G2-XS Qtof mass spectromete. Catalytic activity A typical “the cyclization of propargylamine with CO 2 ” reaction was used to evaluate the catalytic performance of Ag 4 NC. Ag 4 NC (0.4 mg, 0.2×10 −3 mmol), propargylamines (0.5 mmol), and 1,8-Diazabicyclo [5.4.0] undec-7-ene(DBU) (0.05 mmol) were added to acetonitrile (1 mL) in the reaction tube. The reaction stirring for 2 h at 25 °C with the balloon in Carbon dioxide atmosphere. After the reaction stopped, The reaction solution was diluted by dichloromethane, The conversion and selectivity were determined by GC analysis and column chromatography (EtOAc/PE = 1:5).